Wigner and Kondo physics in quantum point contacts revealed by scanning gate microscopy Quantum point contacts exhibit mysterious conductance anomalies in addition to well-known conductance plateaus at multiples of 2 e 2 / h . These 0.7 and zero-bias anomalies have been intensively studied, but their microscopic origin in terms of many-body effects is still highly debated. Here we use the charged tip of a scanning gate microscope to tune in situ the electrostatic potential of the point contact. While sweeping the tip distance, we observe repetitive splittings of the zero-bias anomaly, correlated with simultaneous appearances of the 0.7 anomaly. We interpret this behaviour in terms of alternating equilibrium and non-equilibrium Kondo screenings of different spin states localized in the channel. These alternating Kondo effects point towards the presence of a Wigner crystal containing several charges with different parities. Indeed, simulations show that the electron density in the channel is low enough to reach one-dimensional Wigner crystallization over a size controlled by the tip position. Quantum point contacts (QPCs) [1] are among the simplest quantum devices made out of a two-dimensional electron gas (2DEG). Applying a negative voltage on a split-gate creates a quasi-one-dimensional (1D) channel connected to large 2D reservoirs. This narrow channel behaves as an electron waveguide and transmits a finite number of modes, each of them carrying one quantum of conductance G 0 =2 e 2 / h ( e is the electron charge and h the Planck constant). As a result, the conductance versus gate voltage curve shows a series of quantized plateaus with transitions, which are well reproduced by a single-particle model [2] . However, since the early days of QPCs, a shoulder-like feature is commonly observed [3] at a conductance around 0.7 G 0 , which cannot be explained by single-particle theories. With lowering temperature, this ‘0.7 anomaly’ rises to reach the first plateau, and a zero-bias peak called ‘zero-bias anomaly’ (ZBA) emerges in the non-linear differential conductance [4] . These anomalies have been extensively studied through transport experiments [3] , [4] , [5] , [6] , [7] , revealing the complexity of the underlying phenomena. Different theoretical models have been proposed [8] , [9] , [10] , [11] , [12] , [13] , but no consensus could be reached so far on their interpretation [14] . Recently, an experiment using several gates to vary the channel length [15] revealed the possible existence of several emergent localized states responsible for the conductance anomalies. At the same time, a different theoretical model was proposed [16] , explaining the anomalies without invoking localized states in the channel. As stressed in ref. 17 , investigating these anomalies using scanning probe techniques could make it possible to check the existence of spontaneously localized states and discriminate between these two proposals: this is the aim of the present letter. Here we perform scanning gate microscopy (SGM) [18] , in which a negatively charged tip is scanned above the sample surface and modifies the electrostatic potential in the 2DEG. This local potential change induces electron backscattering towards the QPC, which can be used to image single-particle phenomena such as wave-function quantization in the channel [19] , branched flow in the disorder potential [20] , interference patterns induced by the tip [21] , [22] , [23] , or to investigate electron–electron interactions inside [24] or outside [25] the QPC. This movable gate can also be used to tune in situ the saddle potential of the QPC, in a more flexible and less invasive way than fixed surface gates, and probe intrinsic properties of the QPC such as the 0.7 anomaly [26] , [27] . Here we show that approaching the tip towards the QPC produces an oscillatory splitting of the ZBA, correlated with simultaneous appearances of the 0.7 anomaly, thereby confirming that both features share a common origin [4] , [15] . We interpret these observations as the signature of a small one-dimensional Wigner crystal [28] , [29] , [30] forming in the channel [31] (a quantum chain of charges localized by Coulomb interactions in absence of disorder). The number of charges in this many-body correlated state is tuned by changing the tip position, leading alternatively to a single- or a two-impurity Kondo effect (screening of a localized spin by conducting electrons), with a conductance peak either at zero, or at finite bias, depending on the charge parity. Our observations therefore strongly support the existence of emergent localized states, as suggested in ref. 15 where the number of localized charges is controlled by changing the effective channel length. Here we show that a similar effect is observed when changing the distance of an additional gate placed around the QPC. To understand this new result, we perform classical electrostatic simulations and evaluate the size of the region where electrons should form a 1D Wigner crystal, thanks to the critically low electron density. We show that the calculated size of this small crystal is in good agreement with the observed change in the number of localized charges, thereby revealing that Wigner crystallization is, to our opinion, the correct way to understand this spontaneous localization. Transport measurements The QPC (see Methods and Fig. 1a ) is cooled down to a temperature of 20 mK in a cryogenic scanning probe microscope [32] . In the absence of the tip (moved several microns away), the linear conductance shows the usual staircase behaviour versus gate voltage ( Fig. 1b ). The shoulder below the first quantized plateau is the puzzling 0.7 anomaly. The source-drain bias spectroscopy ( Fig. 1c ) shows that this shoulder evolves to a clear plateau at 0.85 G 0 at finite bias [5] , [33] , [34] . The narrow peak around zero bias is the ZBA and disappears above 1 K ( Supplementary Fig. 1 ). Its width of 200 μeV is much smaller than the 1D subband spacing of 4.5 meV ( Fig. 1d ). Above 0.7 G 0 , the ZBA splits into finite-bias peaks [15] , [35] centred at ±250 μV. We show in the following that the presence of the 0.7 anomaly is related to this splitting of the ZBA. 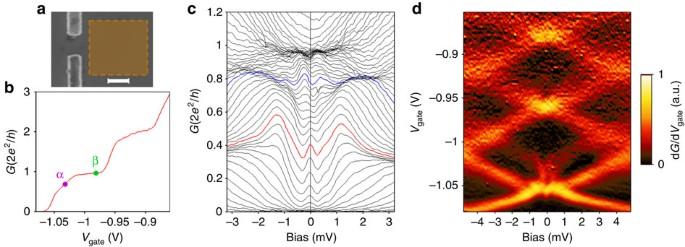Figure 1: Transport measurements. Base temperature is 20 mK. (a) Electron micrograph of the QPC gates. Scale bar, 300 nm. The dashed box indicates the position of the scanning area used inFig. 2. (b) Differential conductanceGat zero bias versus split-gate voltageVgate. The 0.7 anomaly is visible below the first plateau. Positionsαandβare used inFig. 2a,b. (c) Differential conductanceGversus source-drain bias for different gate voltageVgatefrom −1.08 to −0.96 V. The zero-bias peak in the red curve splits into finite-bias peaks in the blue curve. (d) Numerical derivative of the differential conductance dG/dVgateversus bias and gate voltage. Yellow lines highlight transitions between conductance plateaus. Figure 1: Transport measurements. Base temperature is 20 mK. ( a ) Electron micrograph of the QPC gates. Scale bar, 300 nm. The dashed box indicates the position of the scanning area used in Fig. 2 . ( b ) Differential conductance G at zero bias versus split-gate voltage V gate . The 0.7 anomaly is visible below the first plateau. Positions α and β are used in Fig. 2a,b . ( c ) Differential conductance G versus source-drain bias for different gate voltage V gate from −1.08 to −0.96 V. The zero-bias peak in the red curve splits into finite-bias peaks in the blue curve. ( d ) Numerical derivative of the differential conductance d G /d V gate versus bias and gate voltage. Yellow lines highlight transitions between conductance plateaus. Full size image Scanning gate microscopy When the tip is scanned near the QPC and polarized such as to deplete locally the 2DEG (see Methods), we observe two distinct phenomena. On the first conductance plateau ( Fig. 2b ), SGM images reveal the electron flow coming out of the QPC, with fringes spaced by half the Fermi wavelength, as already observed by several groups [20] , [22] , [23] . The fringes result from interferences of electrons backscattered by the depleted region below the tip and reflected by impurities [20] , [22] in the 2DEG or directly by the gates [21] , [36] . 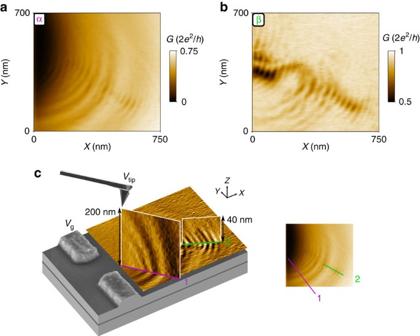Figure 2: Scanning gate microscopy. Base temperature is 20 mK. (a,b) SGM maps of the QPC conductanceGversus tip position in the (X,Y) horizontal plane for gate voltagesVgate=−1 V (a) and −0.95 V (b) corresponding, respectively, to pointsαandβas defined inFig. 1b(gate voltages are shifted by 35 mV in presence of the tip). Concentric rings are only visible atα, and interference fringes are more contrasted atβ. Additional data are presented inSupplementary Fig. 2. (c) Schematic view of the SGM experiment showing the tip scanning above the 2DEG near the QPC gates and three SGM maps. The horizontal map is the same as ina, but the data have been differentiated with respect to the Y-coordinate to highlight details. The two vertical maps are recorded in planes perpendicular to the surface along the purple line 1 (size 500 × 200 nm, gate voltageα) and the green line 2 (size 250 × 40 nm, gate voltageβ) as indicated on the right image (identical toa). The two vertical maps have been differentiated with respect to their horizontal coordinate to highlight details (raw data are shown inSupplementary Fig. 3). The vertical map along line 1 reveals that the concentric rings visible inaform also rings in the vertical plane, whereas the vertical map along line 2 shows that interference fringes disappear rapidly with the tip-to-surface distance. Figure 2: Scanning gate microscopy. Base temperature is 20 mK. ( a , b ) SGM maps of the QPC conductance G versus tip position in the ( X , Y ) horizontal plane for gate voltages V gate =−1 V ( a ) and −0.95 V ( b ) corresponding, respectively, to points α and β as defined in Fig. 1b (gate voltages are shifted by 35 mV in presence of the tip). Concentric rings are only visible at α , and interference fringes are more contrasted at β . Additional data are presented in Supplementary Fig. 2 . ( c ) Schematic view of the SGM experiment showing the tip scanning above the 2DEG near the QPC gates and three SGM maps. The horizontal map is the same as in a , but the data have been differentiated with respect to the Y-coordinate to highlight details. The two vertical maps are recorded in planes perpendicular to the surface along the purple line 1 (size 500 × 200 nm, gate voltage α ) and the green line 2 (size 250 × 40 nm, gate voltage β ) as indicated on the right image (identical to a ). The two vertical maps have been differentiated with respect to their horizontal coordinate to highlight details (raw data are shown in Supplementary Fig. 3 ). The vertical map along line 1 reveals that the concentric rings visible in a form also rings in the vertical plane, whereas the vertical map along line 2 shows that interference fringes disappear rapidly with the tip-to-surface distance. Full size image Below the first plateau ( Fig. 2a ), SGM maps reveal a novel set of concentric rings centred on the QPC, with a spacing increasing with tip distance (see also Supplementary Fig. 2 ). As opposed to the previous one-particle interference fringes, these new rings are not linked to the electron flow (black region in Fig. 2b ) but extend rather isotropically around the QPC, not only in the horizontal plane but in all three directions of space. This is revealed by scanning the tip in a vertical plane ( Fig. 2c ), unveiling half spheres centred on the QPC (purple line 1). This behaviour contrasts with that of interference fringes (green line 2) that quickly disappear when the tip is scanned >50 nm above the surface (see also Supplementary Fig. 3 ). Interferences indeed require electrons at the Fermi level to be backscattered by a depleted region below the tip, a situation which is only obtained for the tip close enough to the 2DEG (and at low enough temperature to avoid thermal averaging of the interferences). We therefore conclude that the new rings are not interferences but result from a direct tuning of the electrostatic potential in the QPC. The larger ring spacing at larger distances results from the smaller potential changes induced by the tip. Conductance anomalies To demonstrate that these rings correspond to modulations of the conductance anomalies, the tip is scanned along a single line in a region with almost no interference (line 3 in Fig. 3a ) and the QPC parameters (gate and bias voltages) are varied. 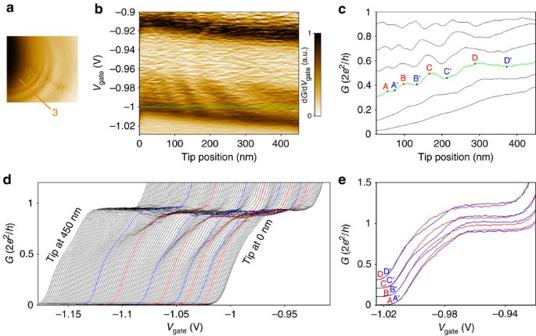Figure 3: Modulation of the 0.7 anomaly. The figure analyses the zero-bias conductance oscillations when the tip is scanned along the orange line 3 indicated inawith the origin of positions in the QPC direction. (b) Trans-conductance dG/dVgateversus tip position and gate voltage. Black regions correspond to transitions between plateaus. The conductance oscillations are only visible below the first plateau. (c) ConductanceGversus tip position for gate voltagesVgate=−0.964, −0.983, −0.992, −1.000, −1.006 and −1.012 V (from top to bottom). Conductance extrema atVgate=−1 V (green curve) are labelled A to D (maxima) and A’ to D’ (minima). The global slope corresponds to the rise of the saddle-point potential when the tip approaches the QPC. (d) ConductanceGversus gate voltage for different tip positions from 0 to 450 nm (successive curves are shifted to the left). (e) Same data as indbut for tip positions A to D (red curves, shifted vertically) and A′ to D′ (blue curves, shifted also horizontally to be compared with red curves). Red curves show no shoulder, whereas blue curves show the 0.7 anomaly. Small differences between plateau values come from residual interference fringes. Figure 3b shows that the ring-related conductance oscillations are only visible for gate voltages in the transition below the first plateau, just where the ZBA and 0.7 anomaly are observed. Figure 3c shows how the conductance oscillations evolve when the average conductance goes from 0 to G 0 while changing the gate voltage. The oscillations are clearly visible between 0.4 and 0.8 G 0 . They are blurred when approaching G 0 because some interference fringes come into play. The increasing distance between conductance extrema (labelled A to D for maxima and A’ to D’ for minima) is consistent with an oscillatory phenomenon in the QPC, controlled by the decreasing electrostatic coupling to the tip. Plotting the conductance versus gate voltage ( Fig. 3d ) reveals the oscillatory behaviour of the 0.7 anomaly. The amplitude of this modulation can be read from Fig. 3e , where curves at positions X and X′ are compared two-by-two (curves are shifted horizontally to compensate for the drift of the pinch-off voltage while approaching the tip). Curves at positions A to D are smooth with no shoulder, that is, no anomaly, whereas curves at positions A′ to D′ present a reduced conductance above 0.5 G 0 , that is, the 0.7 anomaly. The concentric rings observed in SGM images ( Fig. 2a ) therefore correspond to an alternating modulation of the 0.7 anomaly when the tip approaches the QPC. Figure 3: Modulation of the 0.7 anomaly. The figure analyses the zero-bias conductance oscillations when the tip is scanned along the orange line 3 indicated in a with the origin of positions in the QPC direction. ( b ) Trans-conductance d G /d V gate versus tip position and gate voltage. Black regions correspond to transitions between plateaus. The conductance oscillations are only visible below the first plateau. ( c ) Conductance G versus tip position for gate voltages V gate =−0.964, −0.983, −0.992, −1.000, −1.006 and −1.012 V (from top to bottom). Conductance extrema at V gate =−1 V (green curve) are labelled A to D (maxima) and A’ to D’ (minima). The global slope corresponds to the rise of the saddle-point potential when the tip approaches the QPC. ( d ) Conductance G versus gate voltage for different tip positions from 0 to 450 nm (successive curves are shifted to the left). ( e ) Same data as in d but for tip positions A to D (red curves, shifted vertically) and A′ to D′ (blue curves, shifted also horizontally to be compared with red curves). Red curves show no shoulder, whereas blue curves show the 0.7 anomaly. Small differences between plateau values come from residual interference fringes. Full size image We now analyse the behaviour of the ZBA when the 0.7 anomaly repeatedly appears and disappears, and show that both anomalies are linked. 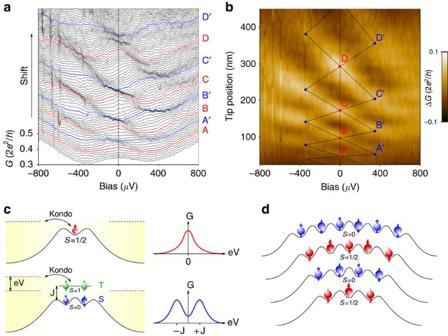Figure 4: Successive splittings of the ZBA. The figure analyses the low bias source-drain spectroscopy when the tip is scanned along the orange line 3 indicated inFig. 3a. (a) Differential conductanceGversus source-drain bias at a fixed gate voltageVgate=−1 V for different tip positions from 0 to 450 nm. Successive curves are shifted upwards by 0.0075 × 2e2/h. Conductance peaks are visible at zero and finite bias on red and blue curves, respectively. (b) Colour plot of the same data as inaafter subtraction of a smooth background to suppress the main gating effect of the tip. Peak positions are indicated by dots. The successive ZBA splittings give a checkerboard pattern. The asymmetry results from the bias-induced change of the QPC position. (c) Schematic of the QPC potential with one (top) and two (bottom) localized electrons, corresponding, respectively, to aS=1/2 ground state with a zero-bias Kondo peak and to aS=0 ground state with finite-bias Kondo peaks involving the excited stateS=1 with singlet-triplet energy splittingJ. The expected conductanceGversus biasVis shown on the right for each state. (d) Schematic of the QPC potential with an increasing number of electrons localized by Coulomb interactions. The antiferromagnetic spin coupling in this small 1D Wigner crystal gives either aS=1/2 ground state (ZBA) or aS=0 ground state (splitting of the ZBA), depending on the parity (respectively odd or even). Figure 4a shows the differential conductance versus source-drain bias for different tip positions (same scan line as in Fig. 3a ). Curves at positions A to D have a peak centred at zero bias (ZBA), whereas curves at positions A′ to D′ have a dip at zero bias and local maxima at ±250 μV bias (splitting of the ZBA), on top of the same V-shaped background. Scanning the SGM tip therefore produces a repetitive splitting of the ZBA, which draws a checkerboard pattern in a colour plot of the spectroscopy versus tip position ( Fig. 4b ). Note that the spontaneous splitting of the ZBA observed without the tip ( Fig. 1c ) also shows peaks at ±250 μV and probably has the same origin. Figure 4: Successive splittings of the ZBA. The figure analyses the low bias source-drain spectroscopy when the tip is scanned along the orange line 3 indicated in Fig. 3a . ( a ) Differential conductance G versus source-drain bias at a fixed gate voltage V gate =−1 V for different tip positions from 0 to 450 nm. Successive curves are shifted upwards by 0.0075 × 2 e 2 / h . Conductance peaks are visible at zero and finite bias on red and blue curves, respectively. ( b ) Colour plot of the same data as in a after subtraction of a smooth background to suppress the main gating effect of the tip. Peak positions are indicated by dots. The successive ZBA splittings give a checkerboard pattern. The asymmetry results from the bias-induced change of the QPC position. ( c ) Schematic of the QPC potential with one (top) and two (bottom) localized electrons, corresponding, respectively, to a S =1/2 ground state with a zero-bias Kondo peak and to a S =0 ground state with finite-bias Kondo peaks involving the excited state S =1 with singlet-triplet energy splitting J . The expected conductance G versus bias V is shown on the right for each state. ( d ) Schematic of the QPC potential with an increasing number of electrons localized by Coulomb interactions. The antiferromagnetic spin coupling in this small 1D Wigner crystal gives either a S =1/2 ground state (ZBA) or a S =0 ground state (splitting of the ZBA), depending on the parity (respectively odd or even). Full size image Considering the regularity of the concentric rings in Fig. 2a , this oscillatory behaviour of the 0.7 and ZBAs would be observed for any scanning line in a large range of angles (see Supplementary Fig. 4 and Supplementary Note 1 ). As a consequence, rings with conductance maxima correspond to a simple staircase in the linear conductance and a ZBA in the non-linear spectroscopy, whereas rings with conductance minima correspond to a 0.7 anomaly and a splitting of the ZBA. This result shows that the ZBA suppresses the 0.7 anomaly at low temperature [4] only if the ZBA is not split into finite-bias peaks. First, we would like to stress again that these new conductance oscillations cannot be explained by interference effects in the 2DEG. One argument already given above is that interferences require backscattering with a tip close to the surface, whereas the new rings are observed up to large tip heights ( Fig. 2c ). A second argument is that interference fringes would have an increasing spacing for short tip distances because the density is reduced close to the QPC and the electron wavelength is larger, but the opposite behaviour is observed. We now discuss a possible single-particle effect inside the QPC that, at first sight, could give similar conductance oscillations. In case of a non-adiabatic transmission, wave functions are scattered by the QPC potential barrier and transmission resonances appear when the barrier length is equal to an integer number of half the longitudinal wavelength. If the effect of the tip is to change the channel length, such resonances could give conductance oscillations versus tip distance. However, this single-particle mechanism cannot explain the repetitive splittings of the ZBA, which are simultaneous with the observed conductance oscillations, and we therefore need another explanation. The ZBA in QPCs has been shown to scale with temperature and magnetic field similar to the Kondo effect in quantum dots [4] . This effect corresponds to the screening of a single degenerate level by a continuum of states, and therefore indicates the presence of a localized spin in the QPC channel [11] . Splittings of the ZBA have been observed recently in length-tunable QPCs [15] and interpreted as a two-impurity Kondo effect [37] , [38] , involving non-equilibrium Kondo screening [39] , [40] , as commonly observed in quantum dots with even numbers of electrons [41] , coupled quantum dots [42] and molecular junctions [43] . We now consider different scenarios to explain the presence of such localized states in our system. In a recent work on QPCs made out of a 2D hole gas, a spontaneous splitting of the ZBA as the QPC opens has been reported [35] . This effect was attributed to a charge impurity forming a potential well close to the channel, containing one or two charges, leading to different types of Kondo screening. In our case, the spontaneous splitting of the ZBA as the QPC opens ( Fig. 1c ) could be explained by this effect. However, the fact that approaching the tip towards the QPC results in four successive splittings of the ZBA indicates that this impurity should contain at least eight charges, which is unlikely for a single impurity. Nevertheless, one could imagine that a shallow quantum dot has formed in the QPC due to potential fluctuations induced by residual disorder [44] and giving Coulomb blockade oscillations as often observed in long 1D wires [45] . The major argument to exclude this scenario is that the split-gate has a larger capacitive coupling to the channel than the tip has (that is, a larger lever-arm parameter), so the split-gate should induce more charging events than the tip, but we observe the opposite: approaching the tip by 600 nm produces four successive splittings of the ZBA and sweeping the gate voltage produces only one splitting. It can therefore not be Coulomb blockade in a disorder-induced quantum dot. The only remaining possibility to explain the presence of localized states in the channel is a spontaneous electron localization, which is not induced by potential barriers but instead by electron–electron interactions. Indeed, a large number of theoretical and numerical investigations show that interactions can localize a finite number of electrons in the channel [12] , [13] , [46] , [47] . On the first conductance plateau and below, transport can be considered as 1D, and the electron density is so low that the Coulomb repulsion overcomes the kinetic energy. When the 1D density n 1D fulfills the criterion n 1 D × a B <1, where a B is the effective Bohr radius (10 nm in GaAs), electrons are expected to spontaneously order in a crystal, with an interparticle distance minimizing Coulomb repulsion [48] . This many-body state, known as a Wigner crystal [28] , [29] , has been suggested to be responsible for the 0.7 anomaly in QPCs [12] . When the electron density in the channel is decreased below the critical value, the density modulations evolve continuously from the λ F /2 periodicity of Friedel oscillations to the λ F /4 periodicity of the Wigner crystal [49] . Quantum Monte Carlo simulations have also shown that electrons in the crystallized region can be relatively decoupled from the high-density reservoirs and present an antiferromagnetic coupling J between adjacent spins [47] . In contrast to the case of quantum dots with real tunnel barriers, electron localization in a QPC is not straightforward and results from emergent barriers in the self-consistent potential. On the other hand, the Kondo effect requires a relatively open system with a good coupling to the reservoirs, and this makes the QPC a suitable platform to observe Kondo phenomena on an interaction-induced localized state, as shown recently in length-tunable QPCs [15] . This last scenario being the most realistic one in our case, we therefore interpret the four observed oscillations as a signature of eight successive states of a small non-uniform 1D Wigner crystal with an alternating odd and even number of localized charges. Situations with an odd number of electrons in a spin S =1/2 ground state show a ZBA due to Kondo screening of non-zero spin states. Situations with an even number of electrons in a spin singlet S =0 ground state show a splitting of the ZBA due to non-equilibrium Kondo screening [39] , [40] of the spin triplet S =1 excited state with peaks at a finite bias eV = J ( Fig. 4c ). The four oscillations, suggestive of eight successive states, reveal that a large number of electrons can spontaneously localize in the channel of a QPC, as shown in Fig. 4d . Observing Kondo screening on a system with many localized charges is not so surprising if we compare with quantum dots where the Kondo effect is observed up to large numbers of electrons [50] . Nevertheless, the particular case of a 1D chain of localized charges in the Kondo regime still requires theoretical investigations. This analysis is consistent with the interpretation given in ref. 15 for similar observations using a QPC with six surface gates to tune the channel length. Our SGM experiment brings additional information on this effect, as scanning the tip around the QPC, laterally or vertically, changes the shape, extension and symmetry of the channel potential. The circular and almost isotropic rings in Fig. 2c show that the localized states survive to all these potential deformations. The regularity of the successive rings also suggests that this localization occurs rather independently of disorder, although possible crystal pinning effects should be investigated in the future. In ref. 15 , the parameter controlling the number of localized states is the effective length of the channel, defined in ref. 51 and computed using an analytical approach assuming a fixed zero potential at the surface [52] . This method is not suitable to model our SGM experiment, as the tip is situated above the surface. To evaluate the potential landscape in the presence of the tip, we perform 3D classical electrostatic simulations in the Thomas–Fermi approximation (see Methods and Supplementary Note 2 ) and compute self-consistently the local potential V ( x , y ) in the 2DEG and the local 2D electronic density n 2D ( x , y ) ( Fig. 5a ). In this way, the tip-induced potential is correctly calculated, with the screening effects from the 2DEG and the metallic gates taken into account. We obtain a good agreement between calculated and experimental values regarding the gate voltage required to close the QPC, the tip voltage to reach depletion in the 2DEG and the cross-talk between the tip position and the QPC opening. The effective channel length used in ref. 15 was calculated in ref. 51 , using the unscreened gate potential. This length cannot be calculated here from our self-consistent potential, because screening effects induce non-parabolic transverse confinement potentials. 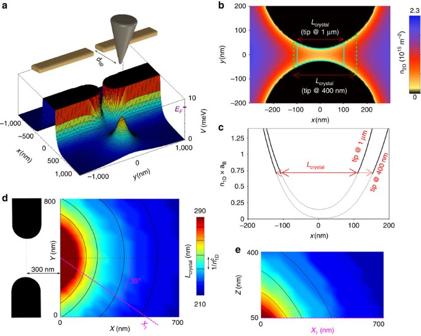Figure 5: Calculation of the electron density and estimation of the Wigner crystal size. (a) Geometry of the metallic gates and SGM tip defined in the Comsol simulation software and example of electrostatic potential map computed for a given gate voltage and tip position. The Fermi energyEFis 8 meV in the 2DEG. (b) Map of the two-dimensional electron densityn2Din the 2DEG computed classically but self-consistently with the potential, when the tip is at 1 μm from the QPC. (c) One-dimensional electron densityn1Dobtained by integration ofn2Dalong theyaxis, when the tip is at 1 μm and 400 nm from the QPC. Choosing a critical densitydetermines the expected sizeLcrystalof the 1D Wigner crystal. (d) Computed size of the Wigner crystal as a function of tip position in an horizontal plane 30 nm above the surface (Vgate=−1 V). The region in red corresponds to a closed contact (the electron density is zero at the QPC center for these tip positions). Black lines indicate tip positions for whichLcrystalis enlarged by, corresponding at first order to the addition of one charge to the crystal. (e) Computed size of the Wigner crystal for tip positions in a vertical plane (above lineX1at 35° from QPC axis). Figure 5: Calculation of the electron density and estimation of the Wigner crystal size. ( a ) Geometry of the metallic gates and SGM tip defined in the Comsol simulation software and example of electrostatic potential map computed for a given gate voltage and tip position. The Fermi energy E F is 8 meV in the 2DEG. ( b ) Map of the two-dimensional electron density n 2D in the 2DEG computed classically but self-consistently with the potential, when the tip is at 1 μm from the QPC. ( c ) One-dimensional electron density n 1D obtained by integration of n 2D along the y axis, when the tip is at 1 μm and 400 nm from the QPC. Choosing a critical density determines the expected size L crystal of the 1D Wigner crystal. ( d ) Computed size of the Wigner crystal as a function of tip position in an horizontal plane 30 nm above the surface ( V gate =−1 V). The region in red corresponds to a closed contact (the electron density is zero at the QPC center for these tip positions). Black lines indicate tip positions for which L crystal is enlarged by , corresponding at first order to the addition of one charge to the crystal. ( e ) Computed size of the Wigner crystal for tip positions in a vertical plane (above line X 1 at 35° from QPC axis). Full size image We propose instead that the parameter controlling the number of localized charges is the size of the region where the 1D Wigner crystallization should occur. This interaction-induced spontaneous ordering is often discussed in terms of the Wigner–Seitz radius r s =1/(2 n 1D a B ), representing the ratio of the Coulomb repulsion to the kinetic energy. A recent numerical investigation of the 1D Wigner crystallization shows that the critical parameter varies between 0.5 and 2, depending on the strength of the transverse confinement potential [48] . To evaluate the size of the region where r s is larger than a given threshold, we calculate the 1D electron density by integration of the 2D electron density in the transverse direction ( Fig. 5b,c ). As an example, we choose a critical value corresponding to a critical density , and evaluate the size L crystal where the density is lower than . This size is found to vary from 210 to 290 nm when the tip is approached by 600 nm towards the QPC, which shows that the tip can strongly affect the size of the low-density region, and hence the number of localized charges. The tip positions leading to the same L crystal form rings centred on the QPC, both for horizontal and vertical scanning planes ( Fig. 5d,e ), in the same way as the conductance oscillations observed in the SGM experiment ( Fig. 2c ). Our classical simulation holds only for an estimate of the size L crystal , but cannot be used to calculate the number of localized charges, as quantum mechanics dominates at such a low density. Note that charges in this crystal are not expected to be uniformly spaced, because the potential of a QPC shows a strong curvature. This non-uniform situation would require an extension of the concept of Wigner crystal, which is usually studied in a flat potential landscape. A rather crude approach to evaluate how many charges can be added by approaching the tip is to suppose that one charge is added to the crystal each time the region is enlarged by (~14 nm for ). With this assumption, approximately five charges can be added to the crystal when the tip is approached close to the QPC ( Fig. 5d ). This value is qualitatively consistent with the four oscillations observed in the experiment, and interpreted as the addition of eight charges. Simulations also show that the number of charges can be modified simply by changing the split-gate voltage (see Supplementary Fig. 5 ). This could explain the ZBA splitting observed above 0.7 G 0 in absence of the tip ( Fig. 1c ). Our assumption that electrons form a 1D system in the low-density region is justified a posteriori by the fact that only the first and second transverse modes are occupied over the length L crystal . The presence of the second mode at the extremities of this region indicates that the system is not strictly 1D, but theory still predicts the formation of a Wigner crystal in the second sub-band of quasi-1D wires, forming a zigzag chain [53] , as possibly observed in experiments [31] , [54] . Interestingly, the simulations show that a small crystallized region survives when the second mode reaches the central part of the channel, which could explain the 0.7 analogues often observed between the first and second conductance plateaus. In summary, we observe a periodic modulation of the conductance anomalies in a QPC at very low temperature while tuning continuously the potential with the polarized tip of a SGM. We explain this experimental observation by the formation of an interaction-induced localized state in the QPC channel, which gives rise to a single- or two-impurity Kondo effect depending on the odd or even number of localized charges, respectively. Indeed, electrostatic simulations show that the electron density in the channel is low enough to result in a spontaneous 1D Wigner crystallization. Our study gives new information on QPC conductance anomalies, which should guide future theoretical works, and will open the way to further experimental investigations involving fine tuning of the QPC potential using various methods. Sample and measurement The QPC is designed on a GaAs/AlGaAs heterostructure hosting a 2DEG 105 nm below the surface with 2.5 × 10 11 cm −2 electron density and 1.0 × 10 6 cm 2 V −1 s −1 electron mobility. A Ti/Au split-gate is defined by e-beam lithography on a mesa with four ohmic contacts and forms a 270-nm-long and 300-nm-wide opening. The device is fixed to the mixing chamber of a dilution fridge, in front of a cryogenic scanning probe microscope [32] , [55] , [56] . The QPC is cooled down to a base temperature of 20 mK at zero gate voltage. The four-probe differential conductance G =d I /d V bias is measured by a standard lock-in technique, using a 10-μV AC excitation at a frequency of 123 Hz. A series resistance of 600 Ω is subtracted from all data to have the conductance of the first plateau at 2 e 2 / h . As the temperature evolution of the zero-bias peak does not saturate below 90 mK, the temperature of electrons in the QPC is probably below this value. Scanning gate microscopy The tip of a commercial platinum-coated cantilever is fixed on a quartz tuning fork, which is mounted on the microscope actuators. The position of the QPC is determined by SGM as the tip position corresponding to the maximum change in conductance while scanning at large tip-surface distance. Next, the tip is lowered to a few tens of nanometres above the surface and scanned at fixed height on a single side of the 200-nm-thick split-gate in the scanning area shown in Fig. 1a . All the SGM results reported here are obtained for a tip voltage of −6 V and a tip-to-surface height of 40 nm (except for vertical scans in Fig. 2c starting at 30 nm). Note that the dilution fridge stays at its base temperature of 20 mK during tip scanning. Electrostatic simulations Classical electrostatic simulations are performed with the Comsol software. We model the system in three dimensions as follows. The 2DEG plane is located 105 nm below the surface according to our heterostructure. The region between the 2DEG and the surface is filled with the GaAs dielectric constant ε r =12.9. The initial electron density in the 2DEG is set at 2.5 × 10 11 e − cm −2 by the addition of a uniform plane of positive charges modelling ionized dopants (in the same plane as the 2DEG for better computation stability). The metallic gates are 120 nm thick and define a 270-nm-wide and 300-nm-long constriction, corresponding to our sample geometry. The tip is modelled by a cone with a 30° full angle and a 30-nm curvature radius at the apex. The tip voltage is fixed at −6 V as in the experiment. For a given choice of gate voltage and tip position, the local potential and density are computed self-consistently by successive iterations. These calculations therefore include screening effects in the 2DEG. How to cite this article: Brun, B. et al. Wigner and Kondo physics in quantum point contacts revealed by scanning gate microscopy. Nat. Commun. 5:4290 doi: 10.1038/ncomms5290 (2014).